High-coverage whole-genome analysis of 1220 cancers reveals hundreds of genes deregulated by rearrangement-mediatedcis-regulatory alterations The impact of somatic structural variants (SVs) on gene expression in cancer is largely unknown. Here, as part of the ICGC/TCGA Pan-Cancer Analysis of Whole Genomes (PCAWG) Consortium, which aggregated whole-genome sequencing data and RNA sequencing from a common set of 1220 cancer cases, we report hundreds of genes for which the presence within 100 kb of an SV breakpoint associates with altered expression. For the majority of these genes, expression increases rather than decreases with corresponding breakpoint events. Up-regulated cancer-associated genes impacted by this phenomenon include TERT , MDM2 , CDK4 , ERBB2 , CD274 , PDCD1LG2 , and IGF2 . TERT -associated breakpoints involve ~3% of cases, most frequently in liver biliary, melanoma, sarcoma, stomach, and kidney cancers. SVs associated with up-regulation of PD1 and PDL1 genes involve ~1% of non-amplified cases. For many genes, SVs are significantly associated with increased numbers or greater proximity of enhancer regulatory elements near the gene. DNA methylation near the promoter is often increased with nearby SV breakpoint, which may involve inactivation of repressor elements. Functionally relevant DNA alterations in cancer extend well beyond exomic boundaries. One notable example of this involves TERT , for which both non-coding somatic point mutations in the promoter or genomic rearrangements in proximity to the gene have been associated with TERT upregulation [1] , [2] , [3] . Genomic rearrangements in cancer are common and often associated with copy number alterations [4] , [5] . Breakpoints associated with rearrangement can potentially alter the regulation of nearby genes, e.g., by disrupting specific regulatory elements or by translocating cis -regulatory elements from elsewhere in the genome into close proximity to the gene. Recent examples of rearrangements leading to “enhancer hijacking”—whereby enhancers from elsewhere in the genome are juxtaposed near genes, leading to overexpression—include a distal GATA2 enhancer being rearranged to ectopically activate EVI1 in leukemia [6] , activation of GFI1 family oncogenes in medulloblastoma [7] , and 5p15.33 rearrangements in neuroblastoma juxtaposing strong enhancer elements to TERT [8] . By integrating somatic copy alterations, gene expression data, and information on topologically associating domains (TADs), a recent pan-cancer study uncovered 18 genes with overexpression resulting from rearrangements of cis -regulatory elements (including enhancer hijacking) [9] . Genomic rearrangement may also disrupt the boundary sites of insulated chromosome neighborhoods, resulting in gene upregulation [10] . The PCAWG Consortium aggregated whole-genome sequencing data from 2658 cancers across 38 tumor types generated by the ICGC and TCGA projects. These sequencing data were reanalyzed with standardized, high-accuracy pipelines to align to the human genome (reference build hs37d5) and identify germline variants and somatically acquired mutations [11] . These data involve a comprehensive and unified identification of somatic substitutions, indels, and structural variants (SVs, representing genomic rearrangement events, each event involving two breakpoints from different genomic coordinates becoming fused together), based on “consensus” calling across three independent algorithmic pipelines, together with initial basic filtering, quality checks, and merging [11] . Whole-genome sequencing offers much better resolution in SV inference over that of whole exome data or SNP arrays [4] , [9] . These data represent an opportunity for us to survey this large cohort of cancers for somatic SVs with breakpoints located in proximity to genes. For a sizeable subset of cases in the PCAWG cohort, data from other platforms in addition to whole-genome sequencing, such as RNA expression or DNA methylation, are available for integrative analyses, with 1220 cases having both whole-genome and RNA sequencing. While SVs can result in two distant genes being brought together to form fusion gene rearrangements (e.g., BCR - ABL1 or TMPRSS2 - ERG ) [12] , this present study focuses on SVs impacting gene regulation in the absence of fusion events or copy number alterations, e.g., SVs with breakpoints occurring upstream or downstream of the gene and involving rearrangement of cis -regulatory elements. In a recent study involving integration of gene expression with low-pass whole-genome sequencing for more than 1000 cancer cases [13] , evidence for a widespread impact of somatic SVs on gene expression patterns was observed, though a noted limitation with that study involved the level of coverage (~6–8×) of low-pass sequencing. With a genome-wide analysis involving a large sample size and much deeper sequencing coverage (~30–60×), information from multiple genes may be leveraged more effectively, in order to identify common features involving the observed disrupted regulation of genes impacted by somatic genomic rearrangement. In this present study, we utilize the PCAWG datasets in order to analyze high coverage whole-genome sequencing data from 1220 individuals. Integrating SV calls with gene expression data, we observe a widespread impact of somatic structural variants on gene expression patterns, independent of copy number alterations, involving key oncogenes and tumor suppressor genes. Mechanisms involved with SV-mediated gene deregulation, as observed here, include enhancer hijacking and altered DNA methylation. Widespread impact of somatic SVs on gene expression Inspired by recent observations in kidney cancer [3] , [14] , neuroblastoma [8] , [15] , and B-cell malignancies [16] , of recurrent genomic rearrangements affecting the chromosomal region proximal to TERT and resulting in its upregulation, we sought to carry out a pan-cancer analysis of all coding genes, for ones appearing similarly affected by somatic rearrangement. We referred to a dataset of somatic SVs called for high coverage whole cancer genomes of 2658 patients, representing more than 20 different cancer types and compiled and harmonized by the PCAWG initiative from 47 previous studies (Supplementary Data 1 ). Gene expression profiles were available for 1220 of the 2658 patients. We set out to systematically look for genes for which the nearby presence of an SV breakpoint could be significantly associated with changes in expression. In addition to the 0–20 kb region upstream of each gene (previously involved with rearrangements near TERT [3] ), we also considered SV breakpoints occurring 20–50 kb upstream of a gene, 50–100 kb upstream of a gene, within a gene body, or 0–20 kb downstream of a gene (Fig. 1a ). (SV breakpoints located within a given gene were not included in the other upstream or downstream SV sets for that same gene.) For each of the above SV groups, we assessed each gene for correlation between associated SV event and expression. As each cancer type as a group would have a distinct molecular signature [17] , and as genomic rearrangements may be involved in copy alterations [4] , [13] , both of these were factored into our analysis, using linear models. Fig. 1: Structural Variant (SV) breakpoints associated with altered expression of nearby genes. a Numbers of SV breakpoints identified as occurring within a gene body, 0–20 kb upstream of a gene, 20–50 kb upstream of a gene, 50–100 kb upstream of a gene, or 0–20 kb downstream of a gene. For each SV set, the breakdown by alteration class is indicated. SVs with breakpoints located within a given gene are not included in the other upstream or downstream SV sets for that same gene. b For each of the SV sets from part ( a ), numbers of significant genes ( p < 0.001, FDR < 4%), showing correlation between expression and associated SV event. Numbers above and below zero point of y -axis denote positively and negatively correlated genes, respectively. Linear regression models also evaluated significant associations when correcting for cancer type (red) and for both cancer type and gene copy number (green). c Heat map of significance patterns for genes from part ( b ) (from the model correcting for both cancer type and gene copy number). Red, significant positive correlation; blue, significant negative correlation; black, not significant ( p > 0.05); gray, not assessed (<3 SV events for given gene in the given genomic region). d Significantly enriched Gene Ontology (GO) terms for genes positively correlated ( p < 0.001 and FDR < 4%) with occurrence of SV upstream of the gene (for either 0–20 kb, 20–50 kb, or 50–100 kb SV sets). P -values by one-sided Fisher’s exact test. e Patterns of SV versus expression for selected gene sets from part ( d ) (telomerase holoenzyme complex, top; eukaryotic translation initiation factor 2B complex, middle; insulin receptor binding, bottom). Differential gene expression patterns relative to the median across sample profiles. See also Supplementary Data 1 , 2 and Supplementary Fig. 1 . Full size image For each of the genomic regions relative to genes that were considered (i.e., genes with at least three samples associated with an SV breakpoint within the given region), we found widespread associations between SV event and expression, after correcting for expression patterns associated with tumor type or copy number (Fig. 1b and Supplementary Fig. 1a and Supplementary Data 2 ). For gene body, 0–20 kb upstream, 20–50 kb upstream, 50–100 kb upstream, and 0–20 kb downstream regions, the numbers of significant genes at p < 0.001 (corresponding to estimated false discovery rates [18] of <4%, Supplementary Data 2 ) were 518, 384, 416, 496, and 302, respectively. For each of these gene sets, many more genes were positively correlated with SV event (i.e., expression was higher when SV breakpoint was present) than were negatively correlated (on the order of 95% versus 5%). Permutation testing of the 0–20 kb upstream dataset (randomly shuffling the SV event profiles and computing correlations with expression 1000 times) indicated that the vast majority of the significant genes observed using the actual dataset would not be explainable by random chance or multiple testing (with permutation results yielding an average of 30 “significant” genes with standard deviation of 5.5, compared with 384 significant genes found for the actual dataset). Without correcting for copy number, even larger numbers of genes with SVs associated with increased expression were found (Fig. 1b ), indicating that many of these SVs would be strongly associated with copy gain. Many of the genes found significant for one SV group were also significant for other SV groups (Fig. 1c ). Tumor purity, tumor ploidy, and total number of SV breakpoints were not found to represent significant confounders (Supplementary Fig. 1b ). High numbers of statistically significant genes were also found when examining regions further upstream or downstream of genes, up to 1 Mb (Supplementary Fig. 1c ). 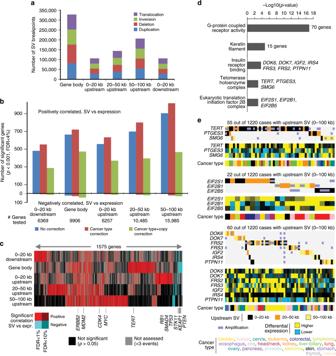Fig. 1: Structural Variant (SV) breakpoints associated with altered expression of nearby genes. aNumbers of SV breakpoints identified as occurring within a gene body, 0–20 kb upstream of a gene, 20–50 kb upstream of a gene, 50–100 kb upstream of a gene, or 0–20 kb downstream of a gene. For each SV set, the breakdown by alteration class is indicated. SVs with breakpoints located within a given gene are not included in the other upstream or downstream SV sets for that same gene.bFor each of the SV sets from part (a), numbers of significant genes (p< 0.001, FDR < 4%), showing correlation between expression and associated SV event. Numbers above and below zero point ofy-axis denote positively and negatively correlated genes, respectively. Linear regression models also evaluated significant associations when correcting for cancer type (red) and for both cancer type and gene copy number (green).cHeat map of significance patterns for genes from part (b) (from the model correcting for both cancer type and gene copy number). Red, significant positive correlation; blue, significant negative correlation; black, not significant (p> 0.05); gray, not assessed (<3 SV events for given gene in the given genomic region).dSignificantly enriched Gene Ontology (GO) terms for genes positively correlated (p< 0.001 and FDR < 4%) with occurrence of SV upstream of the gene (for either 0–20 kb, 20–50 kb, or 50–100 kb SV sets).P-values by one-sided Fisher’s exact test.ePatterns of SV versus expression for selected gene sets from part (d) (telomerase holoenzyme complex, top; eukaryotic translation initiation factor 2B complex, middle; insulin receptor binding, bottom). Differential gene expression patterns relative to the median across sample profiles. See also Supplementary Data1,2and Supplementary Fig.1. Key driver genes in cancer impacted by nearby SV breakpoints Genes with increased expression associated with nearby SV breakpoints included many genes with important roles in cancer (Table 1 ), such as TERT (significant with p < 0.001 for regions from 0–20 kb downstream to 20–50 kb upstream of the gene), MYC (significant for gene body SV breakpoints), MDM2 (regions from 0–20 kb downstream to 50–100 kb upstream), CDK4 (0–20 kb downstream and 20–100 kb upstream), ERBB2 (gene body to 50–100 kb upstream), CD274 (0–20 kb downstream to 50–100 kb upstream), PDCD1LG2 (0–20 kb downstream to 20–50 kb upstream), and IGF2 (0–20 kb downstream and 50–100 kb upstream). Genes with decreased expression associated with SV breakpoints located within the gene included PTEN [19] ( n = 50 cases with an SV breakpoint out of 1220 cases with expression data available), STK11 ( n = 15), KEAP1 ( n = 5), TP53 ( n = 22), RB1 ( n = 55), and SMAD4 ( n = 18), where genomic rearrangement would presumably have a role in disrupting important tumor suppressors; for other genes, SV breakpoints within the gene could potentially impact intronic regulatory elements, or could represent potential fusion events (though in a small fraction of cases) [12] , [13] . Examining the set of genes positively correlated ( p < 0.001, FDR < 4%) with occurrence of SV breakpoint upstream of the gene (for either 0–20 kb, 20–50 kb, or 50–100 kb SV sets), enriched gene categories (Fig. 1d ) included G-protein coupled receptor activity (70 genes), telomerase holoenzyme complex ( TERT , PTGES3 , SMG6 ), eukaryotic translation initiation factor 2B complex ( EIF2S1 , EIF2B1 , EIF2B5 ), keratin filament (15 genes), and insulin receptor binding ( DOK6 , DOK7 , IGF2 , IRS4 , FRS2 , FRS3 , PTPN11 ). When taken together, SVs involving the above categories of genes would potentially impact a substantial fraction of cancer cases, e.g., on the order of 2–5% of cases across various types (Fig. 1e ). Gene amplification events (defined as five or more copies) could be observed for a number of genes associated with SVs, but amplification alone in many cases would not account for the elevated gene expression patterns observed (Fig. 1e ). Table 1 Selected genes positively correlated in expression with occurrence of upstream SV breakpoint. Full size table Translocations involving the region 0–100 kb upstream of TERT were both inter- and intrachromosomal (Fig. 2a and Supplementary Data 3 ) and included 170 SV breakpoints and 84 cancer cases, with the most represented cancer types including liver-biliary ( n = 29 cases), melanoma ( n = 17 cases), sarcoma ( n = 15 cases), and kidney ( n = 9 cases). Most of these SV breakpoints were found within 20 kb of the TERT start site (Fig. 2b ), which represented the region where correlation between SV events and TERT expression was strongest (Fig. 2c, d , p < 1E−14, linear regression model). In neuroblastoma, translocation of enhancer regulatory elements near the promoter was previously associated with TERT upregulation [8] , [15] . Here, in a global analysis, we examined the number of enhancer elements [20] within a 0.5 Mb region upstream of each rearrangement breakpoint occurring in proximity to TERT (for breakpoints where the breakpoint mate was oriented away from TERT ). While for unaltered TERT , 21 enhancer elements are located 0.5 Mb upstream of the gene, on the order of 30 enhancer elements on average were within the 0.5 Mb region adjacent to the TERT SV breakpoint (Fig. 2e ), representing a significant increase ( p < 1E−6, paired t -test). A trend was also observed, by which SV breakpoints closer to the TERT start site were associated with a larger number of enhancer elements (Fig. 2d , p < 0.03, Spearman’s correlation). Fig. 2: SVs associated with TERT and its increased expression. a Circos plot showing all intra- and interchromosomal rearrangements 0–100 kb from the TERT locus. b By cancer type, SV breakpoint locations within the region ~100 kb upstream of TERT . Curved line connects two breakpoints common to the same SV. TERT promoter, CpG Islands, and CTCF and Myc binding sites along the same region are also indicated. c Gene expression levels of TERT corresponding to SVs with breakpoints located in the genomic region 0–20 kb downstream to 100 kb upstream of the gene (116 SV breakpoints involving 47 cases). d Where data available, gene expression levels of TERT corresponding to SVs from part ( b ). Expression levels associated with TERT promoter (PM) mutation are also represented. Median expression for unaltered cases represents cases without TERT alteration (SV, promoter mutation, amplification, viral integration) or MYC amplification. For part ( d ), where multiple SVs were found in the same tumor, the SV breakpoint that was closest to the TERT start site was used for plotting the expression. e Numbers of enhancer elements within a 0.5 Mb region upstream of each rearrangement breakpoint are positioned according to breakpoint location. For unaltered TERT , 21 enhancer elements were 0.5 Mb upstream of the gene. See also Supplementary Data 3 . Full size image Consistent with observations elsewhere [4] , [13] , genomic rearrangements could be associated here with copy alterations for a large number of genes (Fig. 1b ), including genes of particular interest such as TERT and MDM2 (Fig. 3a ). However, copy alteration alone would not account for all observed cases of increased expression in conjunction with SV event. For example, with a number of key genes (including TERT , MDM2 , ERBB2 , CDK4 ), when all amplified cases (i.e., with five or more gene copies) were grouped into a single category, regardless of SV breakpoint occurrence, the remaining SV-involved cases showed significantly increased expression (Fig. 3b ). Regarding TERT in particular, a number of types of genomic alteration may act upon transcription, including upstream SV breakpoint, TERT amplification [21] , promoter mutations [1] , [2] , promoter viral integration [22] , and MYC amplification [23] . Within the PCAWG cohort of 2658 cancer cases, 933 (35%) were altered according to at least one of the above alteration classes, with each class being associated with increased TERT mRNA expression (Fig. 3c ). Upstream SV breakpoints in particular were associated with higher TERT as compared with promoter mutation or amplification events. Fig. 3: SV breakpoints in proximity to key genes uniquely contribute to cases of high expression. a For 1220 cancer cases, copy number versus expression for TERT (left) and MDM2 (right). Cases with SV events upstream of the gene are indicated. 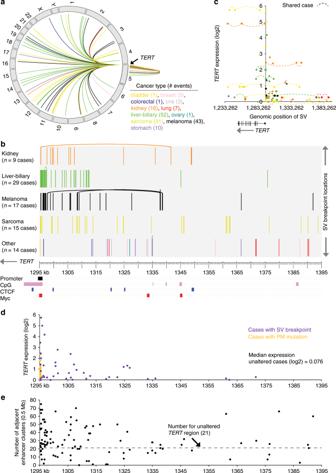Fig. 2: SVs associated withTERTand its increased expression. aCircos plot showing all intra- and interchromosomal rearrangements 0–100 kb from the TERT locus.bBy cancer type, SV breakpoint locations within the region ~100 kb upstream ofTERT. Curved line connects two breakpoints common to the same SV.TERTpromoter, CpG Islands, and CTCF and Myc binding sites along the same region are also indicated.cGene expression levels ofTERTcorresponding to SVs with breakpoints located in the genomic region 0–20 kb downstream to 100 kb upstream of the gene (116 SV breakpoints involving 47 cases).dWhere data available, gene expression levels ofTERTcorresponding to SVs from part (b). Expression levels associated withTERTpromoter (PM) mutation are also represented. Median expression for unaltered cases represents cases withoutTERTalteration (SV, promoter mutation, amplification, viral integration) orMYCamplification. For part (d), where multiple SVs were found in the same tumor, the SV breakpoint that was closest to theTERTstart site was used for plotting the expression.eNumbers of enhancer elements within a 0.5 Mb region upstream of each rearrangement breakpoint are positioned according to breakpoint location. For unalteredTERT, 21 enhancer elements were 0.5 Mb upstream of the gene. See also Supplementary Data3. b Box plots of expression for TERT , MDM2 , ERBB2 , and CDK4 by alteration class (“amp.” or gene amplification: 5 or more copies, SV breakpoint within gene body, SV breakpoint 0–20 kb downstream of gene, SV breakpoint 0–20 kb upstream of gene, SV breakpoint 20–50 kb upstream of gene, SV breakpoint 50–100 kb upstream of gene, or none of the above, i.e., “unaligned”). Cases with both SV breakpoint and amplification are assigned here within the amplification group. Asterisks (“*”) denote statistically significant differences versus unaligned group as indicated. c Left: Alterations involving TERT (SV breakpoint 0–50 kb upstream of gene, somatic mutation in promoter, viral integration within TERT promoter, 5 or more gene copies of TERT or MYC ) found in the set of 1220 cancers cases having both whole-genome sequencing and RNA data available. Right: Box plot of TERT expression by alteration class. “TERT amp” group does not include cases with other TERT -related alterations (SV, Single Nucleotide Variant or “SNV”, viral). P -values by Mann–Whitney U-test; “*” denotes significant differences versus unaligned group with p < = 0.002, and “**” denotes significant differences with p < 1E−6. n.s., not significant ( p > 0.05). Box plots represent 5, 25, 50, 75, and 95%. Points in box plots are colored according to tumor type as indicated in part ( c ). Full size image SVs associated with CD274 (PD1) and PDCD1LG2 (PDL1)—genes with important roles in the immune checkpoint pathway—were associated with increased expression of these genes (Fig. 4a and Supplementary Data 4 ). Out of the 1220 cases with gene expression data, 19 harbored an SV breakpoint in the region involving the two genes, both of which reside on chromosome 9 in proximity to each other (Fig. 4b , considering the region 50 kb upstream of CD274 to 20 kb downstream of PDCD1LG2 ). These 19 cases included lymphoma ( n = 5), lung (4), breast (2), head and neck (2), stomach (2), colorectal (1), and sarcoma (1). Six of the 19 cases had amplification of one or both genes, though on average cases with associated SV had higher expression than cases with amplification but no SV breakpoint (Fig. 4a , p < 0.0001 t -test on log-transformed data). For most of the 19 cases, the SV breakpoint was located within the boundaries of one of the genes (Fig. 4a ), while both genes tended to be elevated together regardless of the SV breakpoint position (Fig. 4b ). We examined the 19 cases with associated SVs for fusions involving either CD274 or PDCD1LG2 , and we identified a putative fusion transcript for RNF38 -> PDCD1LG2 involving three cases, all of which were lymphoma. No fusions were identified involving CD274 . Fig. 4: SVs associated with PD1/PDL1 genes and their increased expression. a Patterns of SV, gene amplification (5 or more copies), RNF38 -> PDCD1LG2 gene fusion, and differential expression for CD274 (PD1 gene) and PDCD1LG2 (PDL1 gene), for the subset of cases with associated SV or amplification for either gene. Differential gene expression patterns relative to the median across sample profiles. b Gene expression levels of CD274 and of PDCD1LG2 , corresponding to the position of SV breakpoints located in the surrounding genomic region on chromosome 9 (representing 66 SV breakpoints involving 19 cases). Median expression for unaltered cases represents cases without SV or amplification. See also Supplementary Data 4 . Full size image Translocated enhancers and altered DNA methylation Similar to analyses focusing on TERT (Fig. 2d ), we examined SVs involving other genes for potential translocation of enhancer elements. For example, like TERT , SVs with breakpoints 0–20 kb upstream of CDK4 were associated with an increased number of upstream enhancer elements as compared with that of the unaltered gene (Fig. 5a ); however, SV breakpoints upstream of MDM2 were associated with significantly fewer enhancer elements compared with that of the unaltered region (Fig. 5a ). For the set of 1233 genes with at least 7 SV breakpoints 0–20 kb upstream and with breakpoint mate on the distal side from the gene, the numbers of enhancer elements 0.5 Mb region upstream of rearrangement breakpoints was compared with the number for the unaltered gene (Fig. 5b and Supplementary Data 5 ). Of these genes, 24% showed differences at a significance level of p < 0.01 (paired t -test, with ~12 nominally significant genes being expected by chance, FDR = 4%). However, for most of these genes, the numbers of enhancer elements was decreased on average with the SV breakpoint rather than increased (195 versus 103 genes, respectively), indicating that translocation of greater numbers of enhancers might help explain the observed upregulation for some but not all genes. For other genes (e.g., HOXA13 and CCNE1 ), enhancer elements on average were positioned in closer proximity to the gene as a result of the genomic rearrangement (Fig. 5c ). Of 829 genes examined (with at least 5 SV breakpoints 0–20 kb upstream and with breakpoint mate on the distal side from the gene, where the breakpoint occurs between the gene start site and its nearest enhancer in the unaltered scenario), 8.3% showed a significant decrease ( p < 0.01, paired t -test, FDR = 10.8%) in distance to the closest enhancer on average as a result of the SV breakpoint, as compared with 1% showing a significance increase in distance. Fig. 5: Translocation of enhancer elements associated with SV breakpoints near genes. a For TERT , ERBB2 , CDK4 , and MDM2 , average number of enhancer elements within a 0.5 Mb region upstream of each rearrangement breakpoint (considering the respective SV sets occurring 0–20 kb upstream of each gene), as compared with the number of enhancers for the unaltered gene. All differences are significant with p < 0.01 (paired t -test). Error bars denote standard error. b For 1233 genes with at least 7 SV breakpoints 0–20 kb upstream and with breakpoint mate on the distal side from the gene, histogram of t -statistics (paired t -test) comparing numbers of enhancer elements 0.5 Mb region upstream of rearrangement breakpoints with the number for the unaltered gene. Positive versus negative t -statistics denote greater versus fewer enhancers, respectively, associated with the SVs. c For 829 genes (with at least 5 SV breakpoints 0–20 kb upstream and with breakpoint mate on the distal side from the gene, where the breakpoint occurs between the gene start site and its nearest enhancer in the unaltered scenario), histogram of t -statistics (paired t -test) comparing the distance of the closest enhancer element upstream of rearrangement breakpoints with the distance for the unaltered gene. Negative t -statistics denote a shorter distance associated with the SV breakpoints. See also Supplementary Data 5 . Full size image We went on to examine genes impacted by nearby SV breakpoints for associated patterns of DNA methylation. Taking the entire set of 8256 genes with associated CpG island probes represented on the 27K DNA methylation array platform (available for samples from The Cancer Genome Atlas), the expected overall trend [24] of inverse correlations between DNA methylation and gene expression were observed (Fig. 6a and Supplementary Fig. 2 and Supplementary Data 6 ). 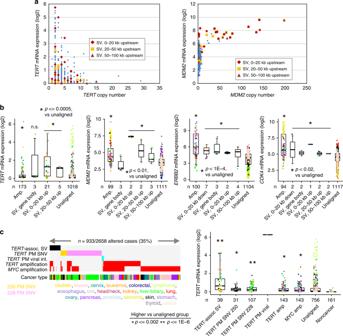Fig. 3: SV breakpoints in proximity to key genes uniquely contribute to cases of high expression. aFor 1220 cancer cases, copy number versus expression forTERT(left) andMDM2(right). Cases with SV events upstream of the gene are indicated.bBox plots of expression forTERT,MDM2,ERBB2, andCDK4by alteration class (“amp.” or gene amplification: 5 or more copies, SV breakpoint within gene body, SV breakpoint 0–20 kb downstream of gene, SV breakpoint 0–20 kb upstream of gene, SV breakpoint 20–50 kb upstream of gene, SV breakpoint 50–100 kb upstream of gene, or none of the above, i.e., “unaligned”). Cases with both SV breakpoint and amplification are assigned here within the amplification group. Asterisks (“*”) denote statistically significant differences versus unaligned group as indicated.cLeft: Alterations involvingTERT(SV breakpoint 0–50 kb upstream of gene, somatic mutation in promoter, viral integration withinTERTpromoter, 5 or more gene copies ofTERTorMYC) found in the set of 1220 cancers cases having both whole-genome sequencing and RNA data available. Right: Box plot ofTERTexpression by alteration class. “TERT amp” group does not include cases with otherTERT-related alterations (SV, Single Nucleotide Variant or “SNV”, viral).P-values by Mann–Whitney U-test; “*” denotes significant differences versus unaligned group withp< = 0.002, and “**” denotes significant differences withp< 1E−6. n.s., not significant (p> 0.05). Box plots represent 5, 25, 50, 75, and 95%. Points in box plots are colored according to tumor type as indicated in part (c). However, for the subset of 263 genes positively correlated in expression with occurrence of upstream SV breakpoint ( p < 0.001 and FDR < 4%, 0–20 kb, 20–50 kb, or 50–100 kb SV sets), the methylation-expression correlations were less skewed toward negative ( p = 0.0001 by t -test, comparing the two sets of correlation distributions in Fig. 5a ). Genes positively correlated between expression and methylation included TERT and MDM2 , with many of the same genes also showing a positive correlation between DNA methylation and nearby SV breakpoint (Fig. 6a ). Regarding TERT , a CpG site located in close proximity to its core promotor is known to contain a repressive element [8] , [25] ; non-methylation results in the opening of CTCF binding sites and the transcriptional repression of TERT [25] . In the PCAWG cohort, SV breakpoints occurring 0–20 kb upstream of the gene were associated with increased CpG island methylation (Fig. 6b ), while SV breakpoints 20–50 kb upstream were not; TERT promoter mutation was also associated with increased methylation (Fig. 6c ). Fig. 6: Altered DNA methylation patterns associated with SV breakpoints near genes. a Histogram of t -statistics for correlation between gene expression and DNA methylation (by Pearson’s using log-transformed expression and logit-transformed methylation), for both the entire set of 8256 genes (blue) associated with CpG islands represented on DNA methylation array platform and the subset of 263 genes (red) on methylation platform and positively correlated in expression ( p < 0.001 and FDR < 4%, “OE” for “overexpressed”) with occurrence of upstream SV breakpoint (for either 0–20 kb, 20–50 kb, or 50–100 kb SV sets). b Histogram of t -statistics for correlation between gene expression and SV event (by Pearson’s using logit-transformed methylation), for both the entire set of 2316 genes (blue) with at least three cases with SV breakpoints 0–20 kb upstream and represented on methylation platform and the subset of 97 genes (red) on methylation platform and positively correlated in expression ( p < 0.001 and FDR < 4%) with occurrence of SV breakpoint 0–20 kb upstream. c DNA methylation of the CpG site cg02545192 proximal to the TERT core promoter in cases with SV breakpoint 0–20 kb or 20–50 kb upstream of TERT, in cases with TERT promoter (PM) activation mutation (SNV), in cases with TERT amplification (“amp.”), and in the rest of cases (unaligned). P -values by t -test on logit-transformed methylation beta values; “*” denotes significant differences versus unaligned group with p < = 0.0001. Box plots represent 5, 25, 50, 75, and 95%. Points in box plots are colored according to tumor type as indicated. See also Supplementary Data 6 and Supplementary Fig. 2 . Full size image Using a unique dataset of high coverage whole-genome sequencing and gene expression on tumors from a large number of patients and involving a wide range of cancer types, we have shown here how genomic rearrangement of regions nearby genes, leading to gene upregulation—a phenomenon previously observed for individual genes such as TERT —globally impacts a large proportion of genes and of cancer cases. Genomic rearrangements involved with upregulation of TERT in particular have furthermore been shown here to involve a wide range of cancer types, expanded from previous observations made in individual cancer types such as kidney chromophobe and neuroblastoma. While many of the genes impacted by genomic rearrangement in this present study likely represent passengers rather than drivers of the disease, many other genes with canonically established roles in cancer would be impacted. Outside information can be brought to bear in distinguishing driver from passenger genes, including significant mutation or copy number alteration patterns [26] , [27] , experimental data, and domain-specific expertise. Though any given gene may not be impacted in a large percentage of cancer cases (the more frequently SV-altered gene TERT involving <3% of cancers surveyed), the multiple genes involved leads to a large cumulative effect in terms of absolute numbers of patients. The impact of somatic genomic rearrangements on altered cis -regulation should therefore be regarded as an important driver mechanism in cancer, alongside that of somatic point mutations, copy number alteration, epigenetic silencing, gene fusions, and germline polymorphisms. Our results have implications for personalized or precision medicine, which tends to be primarily focused on mutations within coding regions. While the role of genomic rearrangements in altering the cis -regulation of specific genes within specific cancer types has been previously observed, our present pan-cancer study demonstrates that this phenomenon is more extensive and impacts a far greater number of genes than may have been previously thought. A recent study by Weischenfeldt et al. [9] , utilizing SNP arrays to estimate SV breakpoints occurring within TADs (which confine physical and regulatory interactions between enhancers and their target promoters), uncovered 18 genes (including TERT and IRS4 ) in pan-cancer analyses and 98 genes (including IGF2 ) in cancer type-specific analyses with overexpression associated with rearrangements involving nearby or surrounding TADs. Our present study using PCAWG datasets identifies hundreds of genes impacted by SV-altered regulation, far more than the Weischenfeldt study. In contrast to the Weischenfeldt study, our study could take advantage of high coverage whole-genome sequencing over SNP arrays, with the former allowing for much better resolution in identifying SVs, including those not associated with copy alterations. In addition, while TADs represent very large genomic regions, often extending over 1 Mb, our study pinpoints SV with breakpoints acting within relatively close distance to the gene, e.g., within 20 kb for many genes. In principle, genomic rearrangements could impact a number of regulatory mechanisms, not necessarily limited to enhancer hijacking or TAD disruption, and genes may be altered differently in different samples. The analytical approach of our present study has the advantage of being able to identify robust associations between SVs and expression, without making assumptions as to the specific mechanism. Future efforts can further explore the mechanisms involved with specific genes deregulated by nearby genomic rearrangements. Regarding TERT -associated SVs, for example, previously observed increases in DNA methylation of the affected region had been previously thought to be the result of massive chromatin remodeling brought about by juxtaposition of the TERT locus to strong enhancer elements [8] , which is supported by observations made in this present study involving multiple cancer types. However, not all genes found here to be deregulated by SVs would necessarily follow the same patterns as those of TERT . For example, not all of the affected genes would have repressor elements being inactivated by DNA methylation, and some genes such as MDM2 do not show an increase in enhancer numbers with associated SV breakpoints but do correlate positively between expression and methylation. There is likely no single mechanism that would account for all of the affected genes, though some mechanisms may be common to multiple genes. Integration of other types of information (e.g., other genome annotation features, data from other platforms, or results of functional studies) may be combined with whole-genome sequencing datasets of cancer, in order to gain further insights into the global impact of non-exomic alterations, where the datasets assembled by PCAWG in particular represent a valuable resource. Datasets Datasets of structural variants (SVs), RNA expression, somatic mutation, and copy number were generated as part of the Pan-Cancer Analysis of Whole Genomes (PCAWG) project [11] . The PCAWG workflows are also available as Docker images through Dockstore enabling researchers to replicate the steps involved in the data assembly [11] . In all, 2658 patients with whole-genome data were represented in the PCAWG datasets, spanning a range of cancer types (bladder, sarcoma, breast, liver-biliary, cervix, leukemia, colorectal, lymphoma, prostate, eosophagus, stomach, central nervous system or “cns”, head/neck, kidney, lung, skin, ovary, pancreas, thyroid, uterus). Cancer molecular profiling data were generated through informed consent as part of previously published studies and analyzed in accordance with each original study’s data use guidelines and restrictions. Of the 2658 donors (Supplementary Data 1 ) included among the whitelist (acceptable for all analyses) and graylist (excluded from some analyses carried out as part of PCAWG-led efforts), 1220 had RNA data, 32 of which were graylisted. In accordance with the PCAWG consoritium policy, we included the graylisted cases in our analysis, as these were found to have no issues pertaining to our integration analysis approaches involving RNA and SV data. For SVs, calls were made by three different data centers using different algorithms; calls made by at least two algorithms were used in the downstream analyses, along with additional filtering criteria being used as described by the PCAWG consortium [11] . Somatic SVs were defined by comparison between the tumor and matched normal. The consensus SV calls are available from synapse ( https://www.synapse.org/#!Synapse:syn7596712 ). For copy number, the calls made by the Sanger group using the Ascat NGS algorithm [11] with default parameters were used, which data are available at the ICGC Data Portal (https://dcc.icgc.org/pcawg). Gene copies of five or more were called as amplification events. For somatic mutation of TERT promoter, PCAWG variant calls, as well as any additional data available from the previous individual studies [3] , [11] , [22] , were used (Supplementary Data 1 ). TERT promoter viral integrations were obtained from ref. [22] . 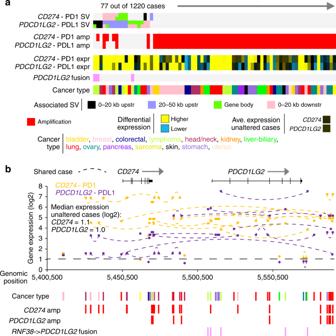Fig. 4: SVs associated with PD1/PDL1 genes and their increased expression. aPatterns of SV, gene amplification (5 or more copies),RNF38->PDCD1LG2gene fusion, and differential expression forCD274(PD1 gene) andPDCD1LG2(PDL1 gene), for the subset of cases with associated SV or amplification for either gene. Differential gene expression patterns relative to the median across sample profiles.bGene expression levels ofCD274and ofPDCD1LG2, corresponding to the position of SV breakpoints located in the surrounding genomic region on chromosome 9 (representing 66 SV breakpoints involving 19 cases). Median expression for unaltered cases represents cases without SV or amplification. See also Supplementary Data4. Of the 2658 cases, RNA-seq data were available for 1220 cases. For RNA-seq data, alignments by both STAR (version 2.4.0i,2-pass) and TopHat2 (version 2.0.12) were used to generated a combined set of expression calls [12] ; alignment parameters and other methodology details are provided at ref. [12] . FPKM-UQ values (where UQ = upper quartile of fragment count to protein coding genes) were used (dataset available at https://www.synapse.org/#!Synapse:syn5553991). Where a patient had multiple tumor sample profiles (this scenario involving a handful of patients), one profile was randomly selected to represent the patient. Overall, RNA-seq samples derived from a similar tissue of origin had similar expression profiles; more specifically, tumor samples from donors derived from different projects were similar and also tissue derived from GTEx versus matched normal tissue were similar, indicating that technical batch effects did not represent a major confounder [12] . In a concerted effort to reduce batch effects due to the use of different computational pipelines in the initial studies, the PCAWG consortium systematically reanalyzed all of the RNA-seq libraries from the individual projects using a unified RNA-seq analysis pipeline, as detailed in ref. [12] . However, it is conceivable that there may be batch effects (e.g., from the isolation and handling of the RNA, library construction and sequencing factors etc.) that have not been possible to take into account. At the same time, where this present study involves integration between orthogonal data platforms, such data integration should be less susceptible to batch effects, as any source of technical variation in one data platform would be less likely to be manifested in the other platform. In addition, our linear models relating SV breakpoint patterns with gene expression (described below) incorporated cancer type as a covariate, and so any genes selected as having significant correlations between SV breakpoints and expression must arise above any associations would be best explained on the basis of cancer type alone. For example, genes that are generally high or low across specific tumor types (whether by biology or by batch effect), irrespective of SV breakpoint pattern, would not be selected as significant. DNA methylation profiles had been generated for 771 cases by The Cancer Genome Atlas using either the Illumina Infinium HumanMethylation450 (HM450) or HumanMethylation27 (HM27) BeadChips (Illumina, San Diego, CA), as previously described [12] . To help correct for batch effects between methylation data platforms (HM450 versus HM27), we used the combat software [12] with R software version 3.0 (with 27K vs 450K as the “batch” and cancer type as the “experimental group”, R code available at https://www.bu.edu/jlab/wp-assets/ComBat/Download_files/ComBat.R), as we have done in previous pan-cancer studies utilizing The Cancer Genome Atlas methylation datasets [14] , [28] , [29] , [30] . For each of 8226 represented genes, an associated methylation array probe mapping to a CpG island was assigned; where multiple probes referred to the same gene, the probe with the highest variation across samples was selected for analysis. Correlations between DNA methylation and gene expression were assessed using logit-transformed methylation data and log-transformed expression data and Pearson’s correlations. Integrative analyses between SVs and gene expression For each of a number of specified genomic region windows in relation to genes, we constructed a somatic SV breakpoint matrix by annotating for every sample the presence or absence of at least one SV breakpoint within the given region. For the set of SV breakpoints associated with a given gene within a specified region in proximity to the gene (e.g., 0–20 kb upstream, 20–50 kb upstream, 50–100 kb upstream, 0–20 kb downstream, or within the gene body), correlation between expression of the gene and the presence of at least one SV breakpoint was assessed using a linear regression model (with log-transformed expression values). In addition to modeling expression as a function of SV event, models incorporating cancer type (one of the 20 major types listed above) as a factor in addition to SV, and models incorporating both cancer type and copy number in addition to SV, were also considered. For these linear regression models, genes with at least three samples associated with an SV breakpoint within the given region were considered. Genes for which SVs were significant ( p < 0.001, FDR < 4%) after correcting for both cancer type and copy were explored in downstream analyses. Results from both the SV only model and results from the SV+cancer type models were also highlighted in Fig. 1 and provided in Supplementary Data 2 , but the p -values from those models were not used in selecting for genes or SVs of interest for follow-up analyses. 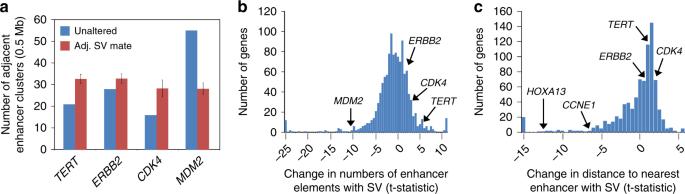Fig. 5: Translocation of enhancer elements associated with SV breakpoints near genes. aForTERT,ERBB2,CDK4, andMDM2, average number of enhancer elements within a 0.5 Mb region upstream of each rearrangement breakpoint (considering the respective SV sets occurring 0–20 kb upstream of each gene), as compared with the number of enhancers for the unaltered gene. All differences are significant withp< 0.01 (pairedt-test). Error bars denote standard error.bFor 1233 genes with at least 7 SV breakpoints 0–20 kb upstream and with breakpoint mate on the distal side from the gene, histogram oft-statistics (pairedt-test) comparing numbers of enhancer elements 0.5 Mb region upstream of rearrangement breakpoints with the number for the unaltered gene. Positive versus negativet-statistics denote greater versus fewer enhancers, respectively, associated with the SVs.cFor 829 genes (with at least 5 SV breakpoints 0–20 kb upstream and with breakpoint mate on the distal side from the gene, where the breakpoint occurs between the gene start site and its nearest enhancer in the unaltered scenario), histogram oft-statistics (pairedt-test) comparing the distance of the closest enhancer element upstream of rearrangement breakpoints with the distance for the unaltered gene. Negativet-statistics denote a shorter distance associated with the SV breakpoints. See also Supplementary Data5. 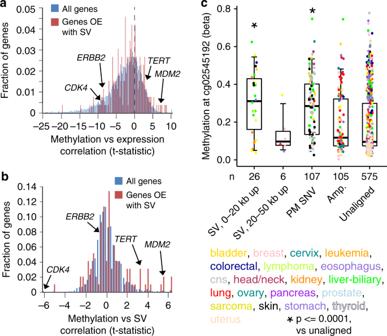Fig. 6: Altered DNA methylation patterns associated with SV breakpoints near genes. aHistogram oft-statistics for correlation between gene expression and DNA methylation (by Pearson’s using log-transformed expression and logit-transformed methylation), for both the entire set of 8256 genes (blue) associated with CpG islands represented on DNA methylation array platform and the subset of 263 genes (red) on methylation platform and positively correlated in expression (p< 0.001 and FDR < 4%, “OE” for “overexpressed”) with occurrence of upstream SV breakpoint (for either 0–20 kb, 20–50 kb, or 50–100 kb SV sets).bHistogram oft-statistics for correlation between gene expression and SV event (by Pearson’s using logit-transformed methylation), for both the entire set of 2316 genes (blue) with at least three cases with SV breakpoints 0–20 kb upstream and represented on methylation platform and the subset of 97 genes (red) on methylation platform and positively correlated in expression (p< 0.001 and FDR < 4%) with occurrence of SV breakpoint 0–20 kb upstream.cDNA methylation of the CpG site cg02545192 proximal to the TERT core promoter in cases with SV breakpoint 0–20 kb or 20–50 kb upstream of TERT, in cases with TERT promoter (PM) activation mutation (SNV), in cases with TERT amplification (“amp.”), and in the rest of cases (unaligned).P-values byt-test on logit-transformed methylation beta values; “*” denotes significant differences versus unaligned group withp< = 0.0001. Box plots represent 5, 25, 50, 75, and 95%. Points in box plots are colored according to tumor type as indicated. See also Supplementary Data6and Supplementary Fig.2. R software version 3.0 and lm function was used, with source code available as part of Supplementary Data 7 . The method of Storey and Tibshirani [18] was used to estimate false discovery rates (FDR) for significant genes. For purposes of FDR, only genes that had SV breakpoints falling within the given region relative to the gene in at least three cases were tested; for example, for the 0–20 kb upstream region, 6257 genes were tested, where 384 genes were significant at a nominal p -value of < 0.001 (using a stringent cutoff, with ~6 genes expected by chance due to multiple testing, or FDR < 2%); the other genomic region windows yielded similar results. For each genomic region window, the FDR for genes significant at the p < 0.001 level did not exceed 4%. In addition, permutation testing of the 0–20 kb upstream dataset was carried out, whereby the SV events were randomly shuffled (by shuffling the patient ids) and the linear regression models (incorporating both cancer type and copy number) were used to compute expression versus permuted SV breakpoint associations; for each of 1000 permutation tests, the number of nominally significant genes at p < 0.001 was computed and compared with results from the actual datasets. Of the 25,259 genes represented in the entire RNA-seq dataset, 20,859 genes had at least three samples with SV breakpoints for at least one of the five regions tested (gene body, 0–20 kb upstream, 20–50 kb upstream, 50–100 kb upstream, 0–20 kb downstream). The number of genes significant (nominal p < 0.001) for any one of the five regions was 1575. By a very conservative estimate, the number of genes that might arise by multiple testing in relation to the 1575 gene set should not exceed 5 × 0.001 × 20859 = 104 (five genomic regions × p -value threshold used × number of genes tested for at least one region), which would correspond to a global estimated FDR of ~6.6%. Integrative analyses using enhancer genomic coordinates Gene boundaries and locations of enhancer elements were obtained from Ensembl (GRCh37 build). Enhancer elements found in multiple cell types (using Ensembl “Multicell” filter, accessed April 1, 2016) were used [20] . As previously described [20] , the Ensembl team first reduced all available experimental data for each cell type into a cell type-specific annotation of the genome; consensus “Multicell” regulatory features of interest, including predicted enhancers, were then defined. For each SV breakpoint 0–20 kb upstream of a gene, the number of enhancer elements near the gene that would be represented by the rearrangement was determined (based on the orientation of the SV breakpoint mate). Only SVs with breakpoints on the distal side from the gene were considered in this analysis; in other words, for genes on the negative strand, the upstream sequence of the breakpoint should be fused relative to the breakpoint coordinates, and for genes on the positive strand, the downstream sequence of the breakpoint (denoted as negative orientation) should be fused relative to the breakpoint coordinates. Statistical analysis All p -values were two-sided unless otherwise specified. Reporting summary Further information on research design is available in the Nature Research Reporting Summary linked to this article.